Bulk magnetoelectricity in the hexagonal manganites and ferrites Improper ferroelectricity (trimerization) in the hexagonal manganites RMnO 3 leads to a network of coupled structural and magnetic vortices that induce domain wall magnetoelectricity and magnetization ( M ), neither of which, however, occurs in the bulk. Here we combine first-principles calculations, group-theoretic techniques and microscopic spin models to show how the trimerization not only induces a polarization ( P ) but also a bulk M and bulk magnetoelectric (ME) effect. This results in the existence of a bulk linear ME vortex structure or a bulk ME coupling such that if P reverses so does M . To measure the predicted ME vortex, we suggest RMnO 3 under large magnetic field. We suggest a family of materials, the hexagonal RFeO 3 ferrites, also display the predicted phenomena in their ground state. Two themes at the forefront of materials physics are the cross-coupling of distinct types of ferroic order [1] , [2] , [3] , [4] and topological defects in systems with spontaneous broken symmetry [5] , [6] , [7] , [8] . Common to both are a plethora of novel phenomenon to understand, and new properties and functionalities to exploit for novel applications. Multiferroics [9] , [10] are an ideal platform to realize both themes in a single material. In this regard, an exciting development is the discovery of a topologically protected vortex domain structure in one of the most extensively studied class of multiferroics, the hexagonal (hexa) rare-earth manganites [11] , [12] , [13] , [14] , [15] . Here, antiphase structural (‘trimer’) domains are clamped to ferroelectric (FE) domain walls (and vice versa) forming a ‘clover-leaf’ pattern ( Fig. 1a ). These trimer domains have a particular phase relationship that result in the appearance of structural vortices, which in turn induce magnetic vortices [16] , [17] , strongly coupled antiferromagnetism and the polarization at the domain wall. This domain wall magnetoelectric (ME) phenomenon produces a magnetization localized at the wall [16] , [17] . 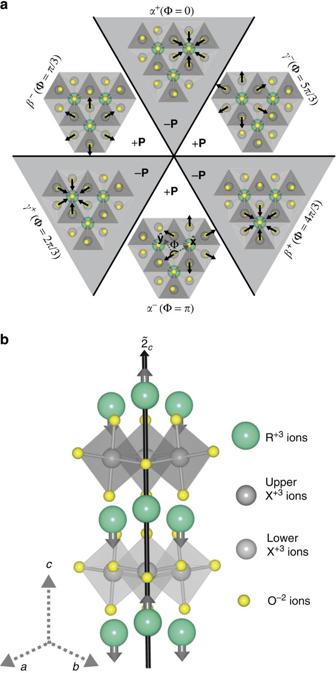Figure 1: Trimer domain and crystal structure. (a) Six structural domains of the ‘trimer’distortion and the polarizationP. Hereα+⇔Φ=0 and a anticlockwise rotation corresponds to domains differing by Φ=+π/3. Arrows indicate the direction of the apical oxygen motion of the trimer distortions, only distortions around theaxis are shown for clarity. (b) FE crystal structure (α+domain). Figure 1: Trimer domain and crystal structure. ( a ) Six structural domains of the ‘trimer’ distortion and the polarization P . Here α + ⇔ Φ=0 and a anticlockwise rotation corresponds to domains differing by Φ=+ π /3. Arrows indicate the direction of the apical oxygen motion of the trimer distortions, only distortions around the axis are shown for clarity. ( b ) FE crystal structure ( α + domain). Full size image The key to realizing these unusual effects is the improper nature of ferroelectricity. Here the polarization P , which is stable in the paraelectric (PE) P6 3 /mmc structure, is induced by a zone-tripling structural distortion, (refs 17 , 18 , 19 ). The latter, referred to as the trimer distortion, is associated with a two-up/one-down buckling of the R -planes and tilting of the MnO 5 bipyramids ( Fig. 1b ). It is nonlinearly coupled to the polarization, the form of which implies that a non-zero trimer distortion induces a non-zero polarization. There are three distinct Φ domains ( α , β and γ ) corresponding to one of the three permutations of two-up/one-down. Moreover, there are two tilting directions, either towards (+) or away (−) from the axis, that is, one-up/two-down or two-up/one-down, respectively. This results in six P6 3 cm structural domains. A consequence of the improper origin of ferroelectricity is that the sign of the polarization depends on the direction of the trimer distortion. This simple fact leads to the non-trivial domain structure of the hexa manganites ( Fig. 1a ) [11] , [12] , [13] , [17] . Recently, thin films of RFeO 3 rare-earth ferrites have been epitaxially stabilized in the hexa manganite P6 3 cm structure [20] , [21] , [22] . This new family of hexa materials exhibit ferroelectricity above room temperature, but with conflicting results as to its origin [23] , [24] . As to the magnetic structure, experiments on LuFeO 3 suggest a considerably high antiferromagnetic (AFM) ordering temperature T N =440 K (ref. 22 ). In addition, there is evidence of a second magnetic transition (~100 K) at which a non-zero magnetization appears [22] , [23] , [24] , [25] , the significance of which, or even if it is an intrinsic or bulk effect, is not known. Our focus here is on elucidating a remarkable interplay of the trimerization, magnetism and polarization in the hexa manganite structure. We show that the trimer structural distortion not only induces a polarization but can also induce both a bulk magnetization and a bulk linear ME effect. This insight leads us to discover bulk phenomena that were not previously seen in a multiferroic, such as the existence of a linear ME vortex structure and a bulk coupling of FE and ferromagnetic domains such that if the polarization reverses 180°, so does the magnetization. We make this clear by connecting an exact microscopic theory of spin–lattice coupling to a simple phenomenological theory, which we test on several hexa manganites and ferrites using first-principles simulation methods. We show that ferroelectricity in the hexa ferrites is of the improper structural type where the trimer distortion induces the polalization, and therefore a similar topological domain structure exists as in the manganites. We explain how the difference in electronic structure between manganites and ferrites requires Fe spins of any hexa ferrite to order in the spin configuration that allows a net magnetization in the ground state. In addition, the much stronger exchange interactions leads to the possibility of spin ordering above room temperature. First-principles calculations on switching Φ by 180° Geometric frustration of the strongly AFM nearest-neighbour (nn) Mn or Fe spins leads to a planar 120° non-collinear order that, because of symmetry, can be described by just two free parameters, Ψ I and Ψ II , even though there are six spins within the unit cell. Note that these reference spins are those connected by the axis that remains in the FE phase, that is, Ψ I ≡Ψ 1 and Ψ II ≡Ψ 2 ( Fig. 2e ). Previously, four principle spin configurations have been denoted as A 1 (− π /2, π /2) ( Fig. 2a ), A 2 ( π ,0) ( Fig. 2c ), B 1 (0,0) ( Fig. 2g ) and B 2 ( π /2, π /2) ( Fig. 2i ). It is well-known that only A 2 (magnetic space group P6 3 c′m′) and intermediate spin configurations that contain a component of A 2 allow a net magnetization along the z axis. What has not been appreciated in the past is that this symmetry-allowed magnetization is in fact induced by the trimer distortion, the consequences of which are quite profound. 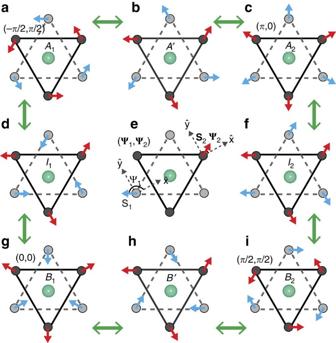Figure 2: Non-collinear spin configurations. Possible 120° spin ordering patterns defined by angles ΨI≡Ψ1and ΨII≡Ψ2(in Φ=0 structural domain). The spin directions are indicated by the blue and red arrows for the magnetic ions in layer I (light grey, small balls) and II (dark grey, small balls), respectively. The centre (large) ball indicates the position of theaxis. The principle configurations, those compatible with crystal symmetry, are denotedA1,A2,B1andB2. OnlyA2and those intermediate configurations that connectA2withA1andB2, denoted asA′ andI2, respectively, allow wFM. Figure 2: Non-collinear spin configurations. Possible 120° spin ordering patterns defined by angles Ψ I ≡Ψ 1 and Ψ II ≡Ψ 2 (in Φ=0 structural domain). The spin directions are indicated by the blue and red arrows for the magnetic ions in layer I (light grey, small balls) and II (dark grey, small balls), respectively. The centre (large) ball indicates the position of the axis. The principle configurations, those compatible with crystal symmetry, are denoted A 1 , A 2 , B 1 and B 2 . Only A 2 and those intermediate configurations that connect A 2 with A 1 and B 2 , denoted as A ′ and I 2 , respectively, allow wFM. Full size image We now begin to make this clear by performing first-principles calculations for two specific examples, LuFeO 3 and LuMnO 3 , in the A 2 phase. Within a typical first-principles calculation of the hexa manganite structure it is easy to reverse the trimer distortion, and hence switch the polarization, via a structural change from a one-up/two-down buckling and tilting ‘in’ of the R -planes and MnO 5 bipyramids, respectively, to a two-up/one-down and tilting ‘out’, thus remaining in the same distinct domain, for example, α + → α − . We perform a series of calculations that follow such a switching path and show these results in Fig. 3 . Our results indicate that the trimer distortion not only induces ferroelectricity but also weak ferromagetism [26] , [27] . 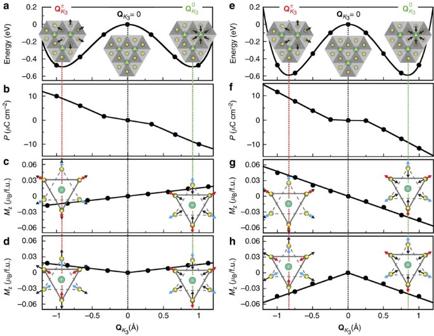Figure 3: First-principles results on switching trimer distortion 180°. Results are shown for LuFeO3(left) and LuMnO3(right). (a,e) Energy as a function of a fixed magnitude of the trimer distortion(no other distortions present), (b,f) polarizationPandc→h, magnetizationM, as a function of a fixed magnitude of. Incandgthe antiferromagnetic spin configuration remains fixed, whereas indandhit rotates 180°. Note that near equilibrium,PandMz, showing thatmediates a bulk linear ME coupling. The fact thatP=0 when=0, indicates that a proper FE mechanism is not likely. This in turn implies that the trimer distortion induces a linear ME effect, Figure 3: First-principles results on switching trimer distortion 180°. Results are shown for LuFeO 3 (left) and LuMnO 3 (right). ( a , e ) Energy as a function of a fixed magnitude of the trimer distortion (no other distortions present), ( b , f ) polarization P and c → h , magnetization M , as a function of a fixed magnitude of . In c and g the antiferromagnetic spin configuration remains fixed, whereas in d and h it rotates 180°. Note that near equilibrium, P and M z , showing that mediates a bulk linear ME coupling. The fact that P =0 when =0, indicates that a proper FE mechanism is not likely. Full size image where E and M are the electric field and magnetization, respectively (see Methods section for derivation). Furthermore, notice that the reversal of the trimer distortion results in one of the two symmetry equivalent situations. In the first case ( Fig. 3c,g ), the AFM configuration remains fixed and the direction of the spin canting reverses (for example, spins cant up rather than down), resulting in the 180° switching of the magnetization. In the second case ( Fig. 3d,h ), the AFM configuration reverses and the spin canting remains fixed, that is, the in-plane component of each spin locally rotates 180°, for example, (Ψ I = π ,Ψ II =0)→(Ψ I =0,Ψ II = π ), resulting in a sign change of the linear ME tensor. These first-principles results are true for all hexa manganites and ferrites in the A 2 phase that we have considered (additional results on ErMnO 3 and ErFeO 3 are given in Supplementary Fig. S1 ) and, as we prove below, is a general property of the A 2 phase. We pause now to stress the point that real switching will occur via a rotation to a neighbouring trimer domain [17] , for example, α + → β − or γ − . These first-principles results, however, contain all of the unique ME physics, that is, if the polarization is reversed, either the bulk magnetization will reverse or the AFM order will change in such a way that the bulk ME tensor changes sign. Route to elucidate cross-coupling of bulk order Our approach to elucidate the bulk, cross-coupling between ferroelectricity and magnetism is to introduce a P6 3 /mmc PE reference structure that has the same AFM configuration as the P6 3 cm FE ground state. The minimal model required to describe the spin structure [28] is the following effective spin Hamiltonian where J ij is the symmetric exchange interactions, D ij is the Dzyaloshinskii–Moriya (DM) antisymmetric exchange vectors and is the single-ion anisotropy (SIA) tensor. Using this model as a guide, we then calculate from first principles how the material-specific parameters of this model change on going from the PE reference structure to the FE ground state as a function of the trimer distortion. This will also allow us to explain why manganites and ferrites have qualitatively different magnetic order. In addition, we will introduce a simple phenomenological model that captures the essential physics, thereby explaining our first-principles results and providing an intuitive rational for the spin model. The magnetic ground state In addition to the four principle magnetic configurations, we also considered the four intermediate non-collinear magnetic structures ( Fig. 2 ). The results of our total energy calculations for LuFeO 3 and LuMnO 3 are presented in Table 1 . In agreement with nonlinear optical measurements [29] , we find that LuMnO 3 stabilizes in the B 1 configuration. This state displays weak antiferromagnetism (wAFM), that is, there is a small canting of the spins out of the x–y plane that leads to a net moment in each layer, but consecutive layers cant in opposite directions, resulting in a net M z =0. Note that the B 2 spin configuration, for which the net magnetic moment in each layer is zero by symmetry, is also close in energy, whereas the A 2 configuration is clearly higher in energy (we point out, however, that A 2 has been stabilized experimentally with the application of a large magnetic field [30] ). Table 1 Non-collinear magnetic energies. Full size table In contrast, we find that LuFeO 3 stabilizes in the A 2 spin configuration. Here the spins also cant out of the x–y plane, but unlike B 1 the net moments in consecutive layers add. This leads to a net M z =0.02 μ B /Fe along the z axis, that is, LuFeO 3 displays weak ferromagnetism (wFM) [26] , [27] . It should be noted that the A 1 ( M z =0 by symmetry) and A ′ (finite M z allowed) configurations lie energetically very close to ground state (we point out that these results are robust with respect to the unknown parameter, U , see Supplementary Table S1 ). Electronic structure In the PE structure, the crystal field at the transition metal (TM) site has a D 3h trigonal point symmetry, which splits the atomic 3 d levels into three sets of states as shown in the insets of Fig. 4 . In the order of increasing energy, these are: e ′ doublet composed of d xz and d yz states, e ′′ doublet composed of d xy and states and singlet that corresponds to state. It is convenient to adopt this notation in the lower symmetry FE phase, even though in this case the crystal field has lower symmetry and the doublets split into singlets. The density-of-states plots calculated for LuFeO 3 and LuMnO 3 in the FE structure are shown in Fig. 4 . LuFeO 3 is a charge-transfer insulator with the conduction band formed by minority Fe 3 d states and the valence band composed of oxygen (O) 2 p states, below which are the filled majority Fe 3 d bands. In LuMnO 3 , the majority 3 d bands are partially filled with occupied e ′ and e ′′. Owing to smaller nuclear charge of Mn, these bands lie at higher energies as compared with LuFeO 3 and they overlap with O 2 p states forming the valence band. At the conduction band minimum we have the empty majority states, whereas minority 3 d levels lie at somehow higher energies. The importance of these differences will be made clear when discussing the magnetic interactions. 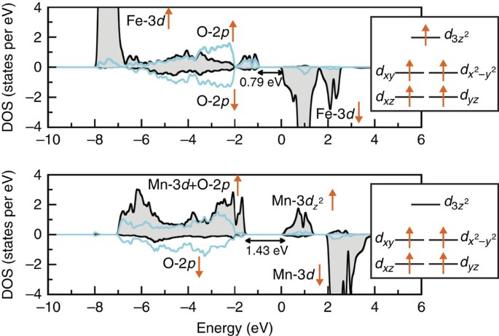Figure 4: The electronic structure from first principles. Density of states (collinear) for LuFeO3(upper panel) and LuMnO3(lower panel) considering the respective magnetic ground state. Note that the difference in orbital occupancy is the fundamental reason why ferrites and manganites have different magnetic ground states, and subsequently the key to the predicted bulk coupling of polarization and magnetism in ferrites. Insets: crystal field splitting and occupancy of the transition metal majority 3dchannel. Figure 4: The electronic structure from first principles. Density of states (collinear) for LuFeO 3 (upper panel) and LuMnO 3 (lower panel) considering the respective magnetic ground state. Note that the difference in orbital occupancy is the fundamental reason why ferrites and manganites have different magnetic ground states, and subsequently the key to the predicted bulk coupling of polarization and magnetism in ferrites. Insets: crystal field splitting and occupancy of the transition metal majority 3 d channel. Full size image Symmetric exchange There are two important symmetric exchange interactions. The first is a strong, AFM superexchange interaction between in-plane, nn spins, J nn . It is much larger in magnitude for LuFeO 3 than for LuMnO 3 (see Supplementary Table S2 ), suggesting a substantially larger magnetic ordering temperature for ferrites (we calculate, within mean field theory, Θ CW =1,525 K and Θ CW =274 K for the Currie–Weiss temperature in the FE phase of LuFeO 3 and LuMnO 3 , respectively (see Supplementary Table S2 )). The second is a weak, super–superexchange interaction, J c , which couples consecutive spin planes via a TM-O-Lu-O-TM exchange pathway, where TM=Fe or Mn ( Supplementary Fig. S2a ). In the PE structure, a spin in one layer is connected to three spins in a consecutive layer. Each of these degenerate spin–spin interactions has two equivalent exchange pathways. We find that the interlayer exchange is AFM for LuFeO 3 but FM for LuMnO 3 . Although the strength of this interaction is relatively weak, this sign difference turns out to be the key. In the PE structure, symmetry implies that the relative orientation of the spins in consecutive spin planes is arbitrary. The trimer distortion, however, splits the three degenerate interactions into (1) a single interaction, mediated by two equivalent TM-O-Lu1-O-TM exchange pathways, and (2) two interactions, where each interaction is mediated by a TM-O-Lu1-O-TM and a TM-O-Lu2-O-TM exchange pathway ( Supplementary Fig. S2b ). Remarkably, this introduces an extra contribution to the energy where Δ J c = , the sign of which is key in determining the spin configuration type: A -type (Ψ II =Ψ I + π ) for Δ J c >0 or B -type (Ψ II =Ψ I ) for Δ J c <0. A simple structural analysis shows that the super–superexchange mediated through the Lu2 ion is always weaker than that mediated through the Lu1 ion, and indeed our calculations show that the magnitude of is always larger than ( Supplementary Table S2 ). We therefore see that the choice between A -type and B -type in the FE structure is in fact determined by the sign of J c in the PE structure. This is important. In ferrites, the AFM nature of the interlayer exchange is uniquely determined by the orbital occupancy, it is always AFM, and therefore ferrites will always prefer A -type magnetic configurations and the wFM ground state (although the interlayer exchange in LuMnO 3 is FM, which explains why it prefers B -type magnetic configurations, it is not universally so; a discussion is given in the Supplementary Note 1 ). DM and SIA Symmetric exchange determines the magnetic configuration type. It is the DM interactions and SIA that drives spin canting (our calculations reveal that a dominant D ij exists only between nn spins within the triangular planes). Let us first consider the PE structure. Here the DM vector has only a component, which favours spin ordering within the x–y plane, whereas the SIA tensor is diagonal with only one independent parameter, τ zz . In the FE structure, however, the trimer distortion induces both a transverse component of the DM vector, , parallel to the x–y plane and an off-diagonal component to the SIA tensor, τ xz . It turns out that these trimer-induced interactions are key and all others can be safely ignored. They lead to a further energy lowering if the spins in each layer, α , cant out of their respective x–y plane. By minimizing equation (3), we find that the canting angle in each layer is for the Φ=0 domain, which vanishes in the PE phase (as xy τ xz =0, where is the strength of the DM interaction). Although this result is easily generalizable to any Φ-domain (see Methods section), next we consider a simple phenomenological model that provides a more intuitive, yet rigorous, generalization and interpretation of our spin-lattice model results. We will clearly show that the trimer-induced exchange interactions are responsible for the bulk polarization–magnetization coupling. The phenomenological model The crystallographic structure suggests that insight may be gained by considering magnetic and structural order parameters (OPs) local to each of the two bipyramid layers. For the magnetic OPs, such consideration is natural. Within each layer ( α =I, II) the local magnetic structure is a combination of 120° AFM order in the x–y plane, L α = L xy , where the angles Ψ I and Ψ II describe the in-plane spin directions of the two reference spins that we previously introduced (and shown again in Fig. 5a for clarity of the present discussion), and a magnetization along the z axis, M α = . To describe the symmetry properties of the former, we introduce a complex OP, L α = . In addition, the layer magnetizations can be represented alternatively by the z components of the total magnetization, M z ≡ /2, and staggered magnetization, L z ≡ /2, per spin. 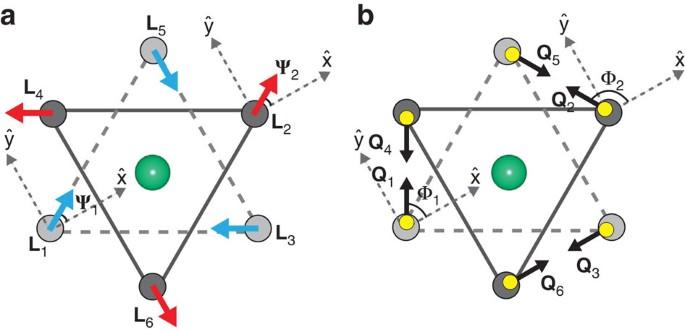Figure 5: In-plane spins and local trimer distortions. (a) The component of theith spin in thex–yplaneLi(i∈1–6). (b) The local trimer distortion at theith siteQi(i∈1–6). We defineLI≡L1andLII≡L2, with spin angles ΨI≡Ψ1and ΨII≡Ψ2, andQI≡Q1andQII≡Q2with local trimer angles ΦI≡Φ1and ΦII≡Φ2. Figure 5: In-plane spins and local trimer distortions. ( a ) The component of the i th spin in the x–y plane L i ( i ∈ 1–6). ( b ) The local trimer distortion at the i th site Q i ( i ∈ 1–6). We define L I ≡ L 1 and L II ≡ L 2 , with spin angles Ψ I ≡Ψ 1 and Ψ II ≡Ψ 2 , and Q I ≡ Q 1 and Q II ≡ Q 2 with local trimer angles Φ I ≡Φ 1 and Φ II ≡Φ 2 . Full size image Following a similar line of reasoning, we describe the total trimer distortion, , as the sum of two local ones, Q α = ( Fig. 5b ). Here we have generalized the suggestion by Artyukhin et al. [17] and defined Φ α as the angle that describes the in-plane displacement of the apical oxygen that lies directly above the reference spin, L α . The complex OP can then be written as . As the relationship Φ 1 = π −Φ 2 ≡ Φ is fixed by the symmetry of the trimer distortion, specific Φ α are associated with the different trimer domains shown in Fig. 1a . Note that a single OP, for example, Q I , fully describes the trimer distortion. The introduction of the second trimer OP, however, allows us to represent the structural distortion in an analogous way as the magnetic ordering. This leads to a particularly transparent form of coupling between structure and magnetism. The transformation properties of the OPs as well as their complex conjugates with respect to symmetry operations of the P6 3 /mmc1′ reference structure are shown in the Supplementary Table S3 . In addition, the transformation properties of a specific combination of these OPs, X η = , are shown where η =±. Note that X η are the only bilinear combinations of the AFM and trimer OPs that are invariant under translation. From this symmetry analysis, it is clear that the following two free-energy invariants are allowed: with denoting the real part. Notice that equation (6) not only contains the spin model result, equation (5), but also generalizes it to any Φ domain. This connection can be made more apparent by defining the vector by Q α = . Then invariants (6) and (7) can be written as whereas the layer magnetization is given by , where and . We can thus interpret as an effective DM vector for layer α . In the Methods section, we generalize the spin–lattice model and arrive at this exact result. This microscopic analysis makes it clear that originates from the transverse component of the DM interaction and off-diagonal elements of the SIA tensor, which are both induced by the trimerization distortion. We verified this point by computing the individual contributions of the DM interaction and the SIA, following the method described in ref. 31 . Writing in terms of local OPs has several conceptual advantages. First, it is immediately clear that in the FE phase canting occurs only when there is a non-zero projection of an x–y spin along the direction of the local trimer distortion, that is, Q α · L α . This is why there is no canting for the A 1 and B 2 spin configurations, as the local spins are perpendicular to the local trimer distortions. In the A 2 and B 1 configurations, however, the local x–y spins and trimer distortions are parallel (or antiparallel), where the only difference being that in A 2 this projection has the same sign in adjacent layers, whereas in B 1 the projection changes sign, resulting in a non-zero and , respectively. As an intermediate spin state can be thought of as a linear combination of principle spin structures, any one with a non-zero A 2 ( B 1 ) component will exhibit wFM (wAFM). Implications of the trilinear coupling The trilinear coupling of equation (6) is quite remarkable. It implies that the trimer distortion not only induces a polarization but also mediates a non-trivial, bulk P – M coupling for any system with A 2 spin ordering. To make this clear, we consider a thought experiment in which an electric field, E , applied along the z axis can switch P to any one of the three trimer domains with − P . Let the system be initially in the α + domain with polarization + P and Q α · L α =−1 ( Fig. 6b ). Next, there are two possible scenarios: { α + → α − } and { α + → β − }. In a proper FE, e.g., PbTiO 3 , the structure of the + P domain is related to the − P domain by a reversal in the direction of the polar distortions with respect to the PE structure, for example, the Ti 4+ ion moving from up to down. The analogous situation in the hexa systems corresponds to a structural change from a one-up/two-down buckling and tilting ‘in’ of the R -planes and bypyramids, respectively, to a two-up/one-down and tilting ‘out’, while remaining in the same distinct domain, for example, α + → α − . This corresponds to switching P via rotating Φ by π ( Fig. 6c ). In this α − domain, because of equation (6), either L α has to rotate 180° ( Q α · L α =−1) or the small canting angle has to change sign ( Q α · L α =+1). It is not unreasonable to expect the latter to be more favourable, leading to a reversal of M . The improper nature of ferroelectricity, however, offers an even more interesting possibility in that there exists three distinct and accessible domains ( α , β and γ ). As an example, let P switch via rotating Φ by π /3 and consider the configuration immediately after ( Fig. 6d ). In this β − domain −1< Q α · L α <0, implying the system is not in equilibrium, and therefore L α must rotate by either | π /3| ( Fig. 6e ) or |2 π /3| ( Fig. 6f ). In the former case Q α · L α =−1 as in the initial α + configuration and, therefore, M is not reversed, whereas in the latter Q α · L α =+1 and M switches 180°. 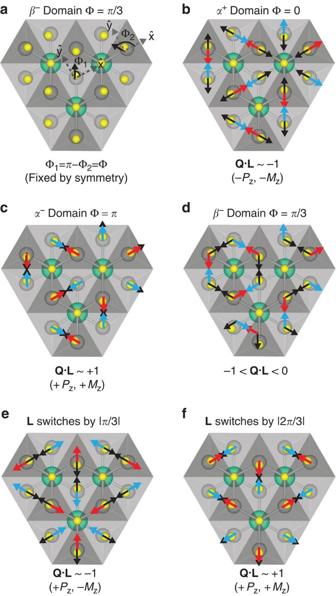Figure 6: Bulk cross-coupling of polarization and magnetization inA2phase. Thought experiment to elucidate the predicted cross-coupling of ferroelectricity and magnetism, mediated by the trimer distortion, withinA2. (a) Definition of local trimer angles ΦIand ΦII(same as inFig. 5b, reproduced here for clarity); (b) Initial equilibriumα+andLdomains. Immediately after switching to the (c)α−domain,Lremains in equilibrium, therefore −Mz→+Mz; (d)β−domain,Lis not in equilibrium and must rotate by either (e) 60°, therefore −Mz→−Mz, or (f) 120°, therefore −Mz→+Mz. Figure 6: Bulk cross-coupling of polarization and magnetization in A 2 phase. Thought experiment to elucidate the predicted cross-coupling of ferroelectricity and magnetism, mediated by the trimer distortion, within A 2 . ( a ) Definition of local trimer angles Φ I and Φ II (same as in Fig. 5b , reproduced here for clarity); ( b ) Initial equilibrium α + and L domains. Immediately after switching to the ( c ) α − domain, L remains in equilibrium, therefore − M z →+ M z ; ( d ) β − domain, L is not in equilibrium and must rotate by either ( e ) 60°, therefore − M z →− M z , or ( f ) 120°, therefore − M z →+ M z . Full size image Having elucidated how the non-polar trimer structural distortion mediates an intrinsic and bulk trilinear coupling of the polarization, magnetization and AFM order, it is natural to ask what type of ME domains would one expect to see. Next, we discuss two probable domain patterns ( Fig. 7 ), but by no means is this meant to be exhaustive. In each case, we assume that the only AFM domain walls present are those clamped to the trimer domain walls [17] . 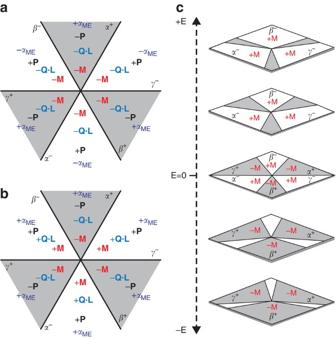Figure 7: Predicted clamping of trimer and magnetic domains and electric field response. At the lowest energy, trimer domain wall Φ changes byπ/3, which will rotate the AFM spin vectors,LIandLII, by either (a)π/3 and −π/3 or (b) −2π/3 and 2π/3. In the former caseMzremains constant, whereas in the latterMzreverses at each trimer domain wall, that is, FE, ferromagnetic and trimer domains are mutually clamped. (c) The schematic diagram displaying the electric-field switching of ferromagnetic domains (note, figure inspired by ref.11). Figure 7: Predicted clamping of trimer and magnetic domains and electric field response. At the lowest energy, trimer domain wall Φ changes by π /3, which will rotate the AFM spin vectors, L I and L II , by either ( a ) π /3 and − π /3 or ( b ) −2 π /3 and 2 π /3. In the former case M z remains constant, whereas in the latter M z reverses at each trimer domain wall, that is, FE, ferromagnetic and trimer domains are mutually clamped. ( c ) The schematic diagram displaying the electric-field switching of ferromagnetic domains (note, figure inspired by ref. 11 ). Full size image Predicted ME domains The first domain configuration ( Fig. 7a ) is such that at trimer domain walls differing by ΔΦ= π /3, for example, at the α + / β − domain wall, the AFM spins rotate ΔΨ I,II =| π /3|. In this case, the direction of the magnetization remains the same across the domain wall, that is, although P switches, M is not reversed, similar to that shown in Fig. 3d,h . Still, there exist a bulk linear ME effect (see Methods section for derivation). This leads to a presence of a remarkable linear ME vortex structure, as the projections, , are equal in all domains, and therefore α zz is of opposite sign in neighbouring trimer domains. The second domain configuration ( Fig. 7b ) is such that at trimer domain walls differing by ΔΦ= π /3, the AFM spins instead rotate by ΔΨ I,II =|2 π /3|. In this case, the magnetization direction reverses with the polarization similar to that shown in Fig. 3c,g . Note that this domain configuration at first appears less likely to be realized than that previously discussed due to a seemingly higher-energy AFM switching pathway. It does, however, provide an avenue for the system to minimize the magnetostatic energy without having to introduce free magnetic domain walls. Indeed, in Fig. 7a there exists a homogeneous magnetization across the entire trimer vortex. In zero field, this has to be unstable towards the formation of ferromagnetic domains. These domain walls can occur within the bulk of a trimer domain, that is, a free AFM domain wall, but there is an energy cost to form this kind of domain wall. An alternative path to minimize the total energy of the system is for the AFM spins to rotate by ΔΨ I,II =|2 π /3| rather than by ΔΨ I,II =| π /3|, thereby alleviating the need to introduce free domain walls. The domain configuration displayed in Fig. 7b is therefore expected whenever the energy to introduce a free AFM domain wall in the bulk of a trimer domain is greater than the energy to rotate the AFM spins by ΔΨ I,II =|2 π /3| rather than by ΔΨ I,II =| π /3|. In Fig. 7c , we sketch the expected response of these domains to electric-field polling. In this process, the positive electric field, E , for example, chooses the (+ P ,+ M ) state, and therefore reversing of the direction of electric field not only switches the direction of polarization but also reverses the direction of magnetization. In the hexa manganites, an A 2 phase can appear under the application of an external magnetic field [30] . As in this case there is a uniform magnetization across the entire trimer vortex, the expected domain configuration is that depicted in Fig. 7a , that is, a linear ME vortex should appear. We have experimentally imaged, using a new technique called ME force microscopy, this predicted ME vortex structure in ErMnO 3 under magnetic field ( Supplementary Fig. S3 ). Here, as the magnetic field is swept from zero to a large (for example) positive value, an ME vortex structure appears as ErMnO 3 enters the A 2 state. Our calculated (from first principles) value of the lattice contribution [32] to the longitudinal linear ME response for ErMnO 3 is α zz =1.04 ps m −1 , which is of the same order of magnitude as the transverse component of Cr 2 O 3 (see Supplementary Fig. S4 and Methods section). The measured value, however, is an order of magnitude greater. Understanding this difference between the measured and the calculated value is an interesting problem that should be further pursued. The ME vortex structure, however, is clearly measurable. In the hexa RFeO 3 materials, the physics that we have discussed can be realized in the ground state. Indeed, our work indicates that ferroelectricity in these materials is of improper structural type where the trimer distortion induces P (see Supplementary Table S5 and Supplementary Fig. S5 ), and therefore a similar topological domain structure exists as in the manganites. The difference in electronic structure between manganites and ferrites, however, requires Fe spins of any hexa ferrite to order in the A 2 spin configuration in ground state. Therefore, both scenarios displayed in Fig. 7 are possible. In addition, the much stronger exchange interactions leads to the possibility of spin ordering above room temperature, as recently suggested by the experiments of ref. 22 . Although unusual for a frustrated magnet, it had been inferred from neutron diffraction [22] that LuFeO 3 orders above room temperature in an AFM state with M =0 and, at a lower temperature, undergoes a re-orientation transition to the A ′ phase inducing a M ≠0. As shown in Table 1 , the A 1 ( M =0 by symmetry) and A ′ (finite M allowed) states lie energetically very close to ground state in LuFeO 3 . Although our calculations are consistent with such a picture, the magnetic ordering in this system at finite temperature needs to be further pursed, but it is clear that the magnetic ground state is A 2 . In this study, we have discussed an intriguing consequence of improper ferroelectricity in the hexa manganite-like systems. We have shown that a non-polar trimer structural distortion not only induces an electrical polarization but also induces bulk wFM, which is a universal feature of A 2 -type hexa systems. This is due to the fact that the trimer distortion mediates an intrinsic bulk trilinear coupling of the polarization, magnetization and AFM order, additionally manifesting in a non-trivial bulk ME effect and domain structure. First-principles calculations The first-principles calculations were performed using the density functional theory+U method [33] with the Perdew-Burke-Ernzerhof (PBE) form of exchange correlation functional [34] . We considered Lu 4 f states in the core, and for TM 3 d states we chose U =4.5 eV and J H =0.95 eV. Structural relaxations, frozen phonon and electric polarization calculations were performed without the spin–orbit coupling using the projector augmented plane-wave basis-based method as implemented in the VASP [35] , [36] . We used a 4 × 4 × 2 k -point mesh and a kinetic energy cut-off value of 500 eV. The Hellman–Feynman forces were converged to 0.001 eV Å −1 . The electronic and magnetic properties were studied in the presence of spin–orbit coupling. We additionally cross-validated the electronic and magnetic properties using the full-potential linear augmented plane wave method as implemented in WIEN2K code [37] . All our calculations were done at 0 K and without applying magnetic or electric filed. The induced DM interaction of a single layer of bipyramids The in-plane, nn DM interactions are mediated by TM-O eq -TM exchange pathways (here O eq denotes an equatorial oxygen atom). In the PE phase, all nn DM vectors are equivalent and only their z components are non-zero. Note that the σ z mirror plane requires DM vectors for adjacent TM–TM bonds to be equal, but opposite in sign (see Fig. 8a ). Physically, this results from a difference in the handedness of the TM-O eq -TM hopping pathways associated with these DM vectors. The z component of the DM vector acts to confine the spins within the x–y plane and does not contribute to canting. We ignored them in the following discussion. In the FE phase, we have two non-equivalent equatorial oxygens: and . Consequently, the nn DM vectors split into two non-equivalent types: one mediated by a TM- -TM path and the other mediated by a TM- -TM path, both of which acquire a non-zero, transverse x–y component that is perpendicular to the corresponding TM–TM bond. Note that a DM vector mediated by a TM- -TM pathway acquires a component parallel to the TM–TM bond (due to different orientations of apical oxygen displacements for the two TM ions). It is expected and confirmed by our first-principles calculations that this component is small and has a minor effect on the TM–TM hopping. In the following, we therefore neglect this parallel component. We point out that inclusion of the parallel component does not change our main conclusions. The transverse components of the DM vectors between TM site 1 and its nn for different trimer domains are shown in Table 2 . 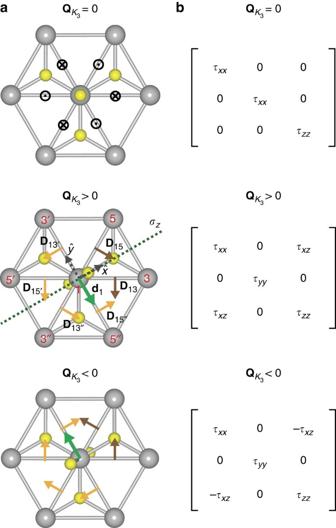Figure 8: DM interactions and SIA. (a) The in-plane nn DM vectors for a single triangular layer of TM ions; (b) SIA tensors for the PE phase and for two opposite directions of the trimer distortion in the FE phase. All six DM vectors acting on TM site 1 and SIA tensor for this site are shown. DM vectors and SIA tensors for other bonds and sites can be generated by applying the appropriate symmetry operations of crystal space group. In the PE phase, only thezcomponent of the nn DM vectors are non-zero, as since triangular layers are mirror planes. The cross (dot) mark represents direction of a DM vector along positive (negative)axis. In the FE structure, the trimer distortion lowers the symmetry, leading to two non-equivalent types of in-plane nn DM vectors: one mediated by TM--TM path and the other mediated by TM--TM path. Figure 8: DM interactions and SIA. ( a ) The in-plane nn DM vectors for a single triangular layer of TM ions; ( b ) SIA tensors for the PE phase and for two opposite directions of the trimer distortion in the FE phase. All six DM vectors acting on TM site 1 and SIA tensor for this site are shown. DM vectors and SIA tensors for other bonds and sites can be generated by applying the appropriate symmetry operations of crystal space group. In the PE phase, only the z component of the nn DM vectors are non-zero, as since triangular layers are mirror planes. The cross (dot) mark represents direction of a DM vector along positive (negative) axis. In the FE structure, the trimer distortion lowers the symmetry, leading to two non-equivalent types of in-plane nn DM vectors: one mediated by TM- -TM path and the other mediated by TM- -TM path. Full size image Table 2 Trimer distortion-induced DM vectors. Full size table Next, we derive the relationship between the local structural distortions and the induced for a single layer α =I. The DM interaction energy (per spin) is given by where by considering Table 2 and/or Fig. 8a we have with . Note that the vectors have equal magnitudes and form a 120° angle with each other. We therefore see a much simpler picture emerging; the relationship between the local structural distortions and the induced DM vectors for an entire layer of bipyramids can be derived by considering a single triangle of spins ( S 1 , S 3 and S 5 ) interacting via ( Fig. 9 ). 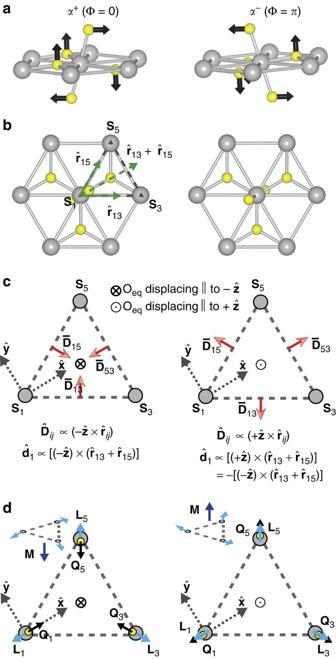Figure 9: Basic ingredients to describe connection between microscopic spin–lattice model and a simple phenomenological model. (a,b) Local trimer distortion aroundS1from two different projections. (c) The transverse components of DM vectors are shown for a single triangle in a single layer. Cross and dot signs denote displacement of the equatorial oxygen alongand, respectively. (d) Relation. Figure 9: Basic ingredients to describe connection between microscopic spin–lattice model and a simple phenomenological model. ( a , b ) Local trimer distortion around S 1 from two different projections. ( c ) The transverse components of DM vectors are shown for a single triangle in a single layer. Cross and dot signs denote displacement of the equatorial oxygen along and , respectively. ( d ) Relation . Full size image As all spins cant in the same direction, we can write S i = L i + M I where L i is the in-plane component of spin S i as previously defined ( Fig. 5 ) and M I is the layer magnetization parallel to the z axis. Substituting this into equation (11), we obtain where the d i are the effective (transverse) DM interactions, for example, d 1 ≡2 . Using A ·( B × C )= B ·( C × A ) and M I = , the DM energy can be rewritten as where the unit vector is defined such that If we assume for the moment that is physically distinct from the DM interaction, we can interpret this relation as saying a induces an effective DM interaction, d i . The question remains whether this is simply a convenient definition to make the analysis look more compact or whether is something new and distinct. To this end, note that it is straightforward to show that a DM vector can be written as (ref. 10 ) where is the displacement of the equatorial oxygen away from the plane ( Fig. 9a ) that arises due to the tilting of the bipyramid and is the unit vector pointing from site i towards j ( Fig. 9b ). Note that in the PE phase the equatorial oxygen is in the x–y plane and therefore U o eq =0. In the FE phase, however, U o eq ± ( Fig. 9c ) and changes sign depending on whether it is in the α + or α − domains. The effective DM vector in the α ± trimer domains can therefore be written as (other d i in the α ± domains can be found by cyclic permutations: 1→3, 3→5 and 5→1), which, considering equation (17), implies and therefore (if we had considered a different domain, for example, β + , the ’s rotate appropriately). It is interesting that is the direction of the in-plane displacement of the apical oxygen that lies directly above spin S i . This is precisely the structural distortion we had chosen to define the local trimer OP (see Fig. 5 ) and first introduced by Mostovoy and coworkers [17] . Furthermore, note that Thus, we obtain which leads to It is becoming clear that the microscopic origin of the layer magnetization is the trimer-induced transverse components of the DM interactions, which cant spins away from the x–y plane. As we will see in the next section, however, there is also another contribution to the canting that originates from the SIA. The SIA of a single layer of bipyramids In the PE phase, the crystal field has the same orientation for all TM ions; thus, the SIA tensor, , does not depend on magnetic site index i . A global coordinate system (see Fig. 8a ) can be thus chosen in which is diagonal with elements τ xx , τ yy and τ zz (see Fig. 8b ). A uniaxial site symmetry and the zero-trace condition lead to τ xx = τ yy =− τ zz /2. On the other hand, in the FE phase the crystal field may have different orientations for different TM ions and therefore does depend on i . Even though all TM ions remain equivalent and thus SIA tensors for different magnetic sites are related by symmetry, in any global coordinate system SIA tensor for some magnetic ions have off-diagonal components. In addition, the uniaxial site symmetry is lost in the FE phase leading to the in-plane anisotropy ( τ xx ≠ τ yy ). In the coordinate system as in Fig. 8a , the SIA tensor for site 1 in the Φ=0 trimer domain is given by For a general trimer domain, the SIA tensor for site 1 is given by where R Φ is a rotation matrix The effect of trimer distortion on the components of the SIA tensor can be understood if we assume that the crystal field for a given TM ion is determined solely by its oxygen bypyramid. In this case, the components of in equation (23) can be expressed in terms of the tilting angle θ and the value of τ zz in the PE phase (hereafter denoted by ). For site 1, we have: First-principles calculations show that the in-plane anisotropy is very small (see Supplementary Table S5 ). Indeed, as seen from equations (25) and (26), this difference is proportional to sin 2 ( θ ), which is a very small quantity. On the other hand, the off-diagonal component, τ xz is proportional to sin(2 θ ), and is correspondingly substantially larger and plays important role in the canting. Let us consider the SIA contribution to the canting energy (per spin) for the layer α =I where we kept only the terms proportional to . The above equation has a similar form as equation (16). Indeed, we can define a DM-like vector as . We then get Energy and magnetization of a single layer of bipyramids Combining equations (16) and (30), we obtain where is the total effective transverse DM vector with strength . Again, using A ·( B × C )= B ·( C × A ) and M I = , E canting can be rewritten as so that the layer magnetization due to canting is given by where J nn is the nn exchange interaction. We thus recovered the result from Landau theory. The stacking of two layers (the real structure) Let us consider now a real hexa structure, which is composed of two layers α =I and α =II, each with a, in principle different, layer magnetization, and , respectively. The canting energy is This can be alternatively written as where M z ≡ and L z ≡ /2 are the total and stagger magnetic moment per spin, respectively. Although the specific sites we choose to define I and II are arbitrary, it is convenient to associate I with site 1 and II with site 2 . As symmetry implies Φ 1 = π −Φ 2 , where Φ 1 (Φ 2 ) is the local trimer angle at site 1 ( 2 ), a single trimer angle, Φ ≡ Φ 1 , can be defined. This single angle was used to define the trimer domains in Fig. 1a . Note that equation (35) is the exact result we derived from Landau theory and explains our first-principles calculations displayed in Fig. 3 ; in the A 2 state, and, therefore, , leading to a net magnetization as we previously showed from first principles. For completeness, note that in the B 1 state, however, the projection has the opposite sign in adjacent layers, . The spins in each plane still cant but as the projection changes sign in adjacent layers no net magnetization exists, . We call this wAFM. The above results can be rewritten in terms of the trimer phase and the spin angles describing wFM for the A 2 phase and wAFM for the B 1 phase, respectively. Phenomenological derivation of linear ME tensor Here we derive the longitudinal component of linear ME susceptibility tensor. The FE phase in the A 2 magnetic structure has P6 3 c′m′ space group. The corresponding point group is 6m′m′, which allows for ME effect with ME susceptibility tensor, To understand the origin of this ME coupling, we consider Landau expansion with respect to the P6 3 /mmc1′ reference structure. The part of the free energy that depends on M z can be written as where we defined . Minimizing with respect to M z , we find an equilibrium magnetization where . Assuming the in-plane spin components are rigid (this assumption is rigorous in the A 2 phase), the zz component of the ME susceptibility is To find ( ∂ Q K 3 ) / ( ∂ E z ) | E z = 0 , we consider the free energy as a function of P z and In the above equation, M z was integrated out resulting in renormalization of the a Q coefficient. Minimizing with respect to P z , we obtain We assume that we are well below the trimerization transition and is large and satisfies >>1. Next, the above equation simplifies to where d p =( d )/( d ′). Minimization of equation (42) with respect to leads to Substituting equation (44) into equation (45), we obtain where , and we took into account that within any trimer domain cos3Φ=±1. Taking derivative with respect to E z at E z =0, we obtain From equation (46), we obtain , leading to Therefore, the ME susceptibility becomes Note that from equations (40) and (44), it follows that Few comments are in order. First, α ∥ is non-zero only when is non-zero, which is exactly the condition for the existence of wFM that requires that the magnetic configuration has a non-zero A 2 component. Second, if is fixed (that is, the projections are equal in all domains), then the sign of α ∥ switches as we go from prime (Φ= π , ± π /3) to non-prime (Φ=0, ±2 π /3) trimer domains. In other words, the domains with parallel M z and P z have an opposite sign of α ∥ than domains with M z and P z antiparallel. Calculation of linear ME tensor from first principles To estimate the value of α zz from equation (49), we calculated numerical values of the parameters used in this equation from first principles. We considered the high-symmetry P6 3 /mmc phase and freezed in the trimer distortion, which corresponds to the zone boundary K 3 mode, then calculated total energy, polarization ( P z ) and magnetic moment ( M z ) per unit cell as a function of the amplitude of the trimer distortion. The a Q parameter was evaluated by fitting the energy versus curve using equation (42) with P z =0. The linear region of the P z versus curve was fitted by the function to evaluate the value of d p and is the slope of the M z ( ) curve. The computed sizes of the parameters d p , a Q , b Q , and and α zz are given in Supplementary Table S6 . We followed the method described in ref. 32 to calculate the lattice linear ME response. We only calculated the longitudinal component α zz of the linear ME susceptibility tensor for one of the specific example, ErMnO 3 . The energy contribution as a function of atomic displacement can be written as where E denotes an external electric field and q n , C n and represent amplitude, eigenvalue of the force–constant matrix and dielectric polarity of the n th mode, respectively. Minimizing equation (51) with respect to q n , we obtain Next, the electric field-induced atomic displacements are given by where e ns represents eigen vector of the n th mode. Thus, we obtain the atomic displacements in the presence of electric field by calculating dielectric polarities, as well as eigen values and vectors of the force–constant matrix at the Γ point of the Brillouin zone of ground state FE P6 3 cm phase. Only infrared active modes contribute to linear ME response. There are ten infrared active modes having A1 symmetry at the Γ that contribute to the change in electric dipole moment along crystallographic z axis. Among them, one is acoustic and nine are optical. We therefore considered these nine infrared active modes and calculated corresponding dielectric polarities, eigen values and vectors (see Supplementary Fig. S4c ). Dielectric polarity is the measure of change in dipole moment with respect to mode amplitude, that is, . The computed linear ME response α zz =(∂ M z )/(∂ E ) (see Supplementary Fig. S4d ) for ErMnO 3 is 1.04 ps m −1 , which is of the same order of magnitude as the transverse component for Cr 2 O 3 and is in good agreement with the estimated value from equation (49) (see Supplementary Table S6 ). How to cite this article: Das, H. et al. Bulk magnetoelectricity in the hexagonal manganites and ferrites. Nat. Commun. 5:2998 doi: 10.1038/ncomms3998 (2014).